Dynamic control of light emission faster than the lifetime limit using VO2phase-change Modulation is a cornerstone of optical communication, and as such, governs the overall speed of data transmission. Currently, the two main strategies for modulating light are direct modulation of the excited emitter population (for example, using semiconductor lasers) and external optical modulation (for example, using Mach–Zehnder interferometers or ring resonators). However, recent advances in nanophotonics offer an alternative approach to control spontaneous emission through modifications to the local density of optical states. Here, by leveraging the phase-change of a vanadium dioxide nanolayer, we demonstrate broadband all-optical direct modulation of 1.5 μm emission from trivalent erbium ions more than three orders of magnitude faster than their excited state lifetime. This proof-of-concept demonstration shows how integration with phase-change materials can transform widespread phosphorescent materials into high-speed optical sources that can be integrated in monolithic nanoscale devices for both free-space and on-chip communication. The tunable properties of phase-change materials provide an exciting opportunity to modulate the optical response of optoelectronic devices, potentially at ultrafast speeds [1] , [2] , [3] , [4] . For example, phase-change materials have been considered as a means to modulate reflection and transmission of nanoscale films and devices [5] , [6] , [7] , [8] . We propose here a new framework to directly modulate light emission from integrated sources faster than their radiative lifetime. The concept is based on the dynamic manipulation of light through tailoring the local density of optical states (LDOS). Such LDOS engineering can be used to control the direction [9] , polarization [10] , [11] and spectrum [12] , [13] of light emission, even at sub-lifetime scales [14] . Here, we use phase-change materials within an engineered optical environment to dynamically control the spontaneous light emission of a quantum emitter. We leverage the ultrafast insulator-to-metal transition (IMT) of vanadium dioxide (VO 2 ) [2] , [3] , [4] as well as the symmetry difference in the polarization of electric dipole (ED) and magnetic dipole (MD) transitions of erbium ions to demonstrate direct all-optical modulation of spontaneous emission at sub-lifetime scales. Distinct from direct ‘electronic’ modulation of off-chip III-V based lasers [15] , [16] , [17] or optical modulation using external interferometers [18] , [19] , [20] , this approach enables both the emitter and modulator to be monolithically integrated into a single nanoscale device. Design The key to realizing optical modulation is to design a multilayer structure such that the phase-change layer can be externally switched by a control laser while also having maximum influence on the LDOS of the emitter layer. A simple design to achieve this goal is a quarter-wavelength phase-change layer (that is, thickness where n is the refractive index) located between an emitter layer and a metal mirror, as shown in Fig. 1a . If the stack is constructed in this way, there is a phase shift in the effective optical path length when the VO 2 is switched from the insulating to metallic state ( Fig. 1b,c ), which maximizes the influence of the phase-change on the surrounding LDOS. 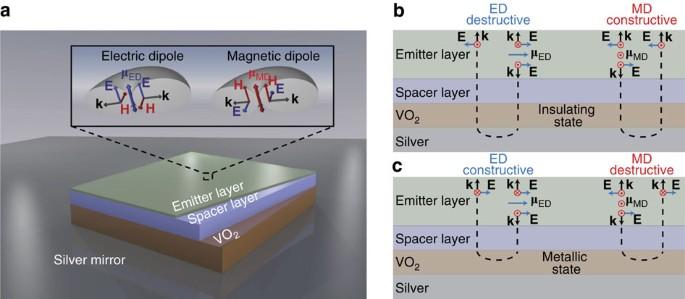Figure 1: Sketch of the sample and illustration of LDOS modulation. (a) Sketch of the sample. Inset shows the polarization symmetries of ED and MD radiation. (b,c) illustrate the interference of ED and MD emission processes when the VO2layer is in the insulating and metallic phases, respectively. Figure 1: Sketch of the sample and illustration of LDOS modulation. ( a ) Sketch of the sample. Inset shows the polarization symmetries of ED and MD radiation. ( b , c ) illustrate the interference of ED and MD emission processes when the VO 2 layer is in the insulating and metallic phases, respectively. Full size image As the process of light emission depends both on the optical environment and on the intrinsic properties of the emitter, engineering spontaneous emission also requires knowledge of the underlying electronic transitions (that is, emission wavelength and dipolar nature). The emission from erbium at 1.5 μm has a multipolar character, showing equal contributions from ED and MD transitions [13] , [21] . Using the energy-momentum spectroscopy set-up shown in Fig. 2a , we can precisely quantify the intrinsic radiative rates of ED and MD transitions in a thin film of Er 3+ :Y 2 O 3 (refs 13 , 22 ; Supplementary Fig. 1 ). The results of this analysis illustrate how the photoluminescence spectrum (shown in Fig. 2b ) originates from a combination of spectrally distinct ED and MD transitions (shown in Fig. 2c ) [13] . These two kinds of transitions typically present differing field symmetries: ED emit with symmetric electric fields, while MD emit with antisymmetric electric fields ( Fig. 1c ). This symmetry difference can be leveraged to dynamically enhance (or suppress) their emission by modifying the electric and magnetic LDOS via the VO 2 IMT and therefore switch between these distinct spectra. 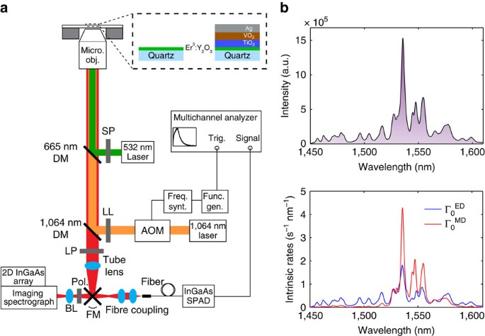Figure 2: Experimental set-up and ED/MD contributions to Er3+emission around 1.5 μm. (a) Experimental set-up used for conventional photoluminescence, energy-momentum spectroscopy and time-resolved measurements. (b) Photoluminescence spectrum of a single-layer Er3+:Y2O3sample. (c) Extracted spectrally resolved intrinsic emission rates for ED (blue) and MD (red) transitions obtained from theoretical fit to experimental energy-momentum spectra (Supplementary Fig. 1). AOM, acousto-optic modulator; BL, Bertrand lens; DM, dichroic mirror; FM, flip mirror; freq. synt., frequency synthesizer; func. gen., function generator; LL, laser line; micro. obj., microscope objective; Pol, polarization; SP, short-pass; SPAD, single-photon avalanche photodiode; trig., trigger. Figure 2: Experimental set-up and ED/MD contributions to Er 3+ emission around 1.5 μm. ( a ) Experimental set-up used for conventional photoluminescence, energy-momentum spectroscopy and time-resolved measurements. ( b ) Photoluminescence spectrum of a single-layer Er 3+ :Y 2 O 3 sample. ( c ) Extracted spectrally resolved intrinsic emission rates for ED (blue) and MD (red) transitions obtained from theoretical fit to experimental energy-momentum spectra ( Supplementary Fig. 1 ). AOM, acousto-optic modulator; BL, Bertrand lens; DM, dichroic mirror; FM, flip mirror; freq. synt., frequency synthesizer; func. gen., function generator; LL, laser line; micro. obj., microscope objective; Pol, polarization; SP, short-pass; SPAD, single-photon avalanche photodiode; trig., trigger. Full size image To this end, we design a multilayer structure ( Fig. 1 ) that comprises an Er 3+ :Y 2 O 3 thin-film emitter, a TiO 2 spacer layer, a VO 2 layer and an Ag mirror. (Expressions for the LDOS in such a five-layer system are explicitly provided in Supplementary Note 1 together with a related schematic in Supplementary Fig. 2 ). 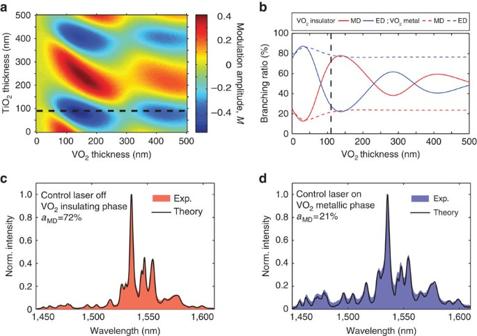Figure 3: Device design and spectral modulation of Er3+emission in multilayer structure. (a) 2D colour plot of the calculated modulation amplitude of the MD contribution to Er3+emission at 1.5 μm upon the VO2phase-change, as a function of TiO2and VO2thicknesses. (b) Evolution of the branching ratio of ED (red) and MD (blue) emission as a function of the VO2thickness (whereas indicated by the black line ina), before (solid lines) and after (dashed lines) inducing the VO2insulator-to-metal transition. The black line labels the VO2thickness used in our experiment. (c,d) Experimental and calculated spectra for Er3+ions when VO2is in the (c) insulating state and (d) metallic state. Experimental spectra are shown in shaded red and blue colour, respectively, whereas theoretically predicted spectra are shown as black solid lines. Exp, experimental; norm, normalized. Figure 3a shows the calculated modulation amplitude of MD emission as a function of the thicknesses of both VO 2 and TiO 2 layers, where and denotes the Er 3+ MD branching ratio for the different phases of VO 2 (more details in Methods section). Figure 3: Device design and spectral modulation of Er 3+ emission in multilayer structure. ( a ) 2D colour plot of the calculated modulation amplitude of the MD contribution to Er 3+ emission at 1.5 μm upon the VO 2 phase-change, as a function of TiO 2 and VO 2 thicknesses. ( b ) Evolution of the branching ratio of ED (red) and MD (blue) emission as a function of the VO 2 thickness (where as indicated by the black line in a ), before (solid lines) and after (dashed lines) inducing the VO 2 insulator-to-metal transition. The black line labels the VO 2 thickness used in our experiment. ( c , d ) Experimental and calculated spectra for Er 3+ ions when VO 2 is in the ( c ) insulating state and ( d ) metallic state. Experimental spectra are shown in shaded red and blue colour, respectively, whereas theoretically predicted spectra are shown as black solid lines. Exp, experimental; norm, normalized. Full size image Switching ED and MD emission using VO 2 As can be seen in Fig. 3a , specific conditions enable the complete reversal of the emission from dominantly MD to dominantly ED (and vice-versa) upon switching of VO 2 . To experimentally investigate this direct modulation of Er 3+ light emission induced by the VO 2 phase-change, we fabricated a multilayer structure with and . For this particular geometry, the device is designed such that the emitter layer has a high magnetic LDOS when VO 2 is in the insulating state, but switches to a high electric LDOS when VO 2 is in the metallic state as shown in Fig. 3b . The shaded curve in Fig. 3c shows the measured spectrum of the sample when continuously pumped by a 532 nm laser. As expected, the spectrum resembles that of dominantly MD emission (as can be seen by comparison to the intrinsic MD rate in Fig. 2c ). Then, using a 1,064 nm control beam, we independently trigger the VO 2 phase-change and demonstrate all-optical modulation of the local optical environment as well as the resulting emission. (Note that the 1,064 nm control laser is chosen to be non-resonant with any Er 3+ transitions). Figure 3d shows the resulting Er 3+ emission spectrum under illumination by both the 1,064 nm control laser and 532 nm pump laser and we see a clear difference in the resulting spectrum. As compared with Fig. 3c , the spectra in Fig. 3d shows the rise of distinct emission peaks between 1,450 and 1,520 nm, which indicates a switch from dominantly MD emission to dominantly ED emission (more details in the Supplementary Fig. 3 ). This is more clearly evidenced in Fig. 4a where the experimental Er 3+ spectra obtained for insulating and metallic VO 2 are displayed together. In addition, when the 1,064 nm laser control beam is turned back off, the Er 3+ emission returns to its initial spectral shape. 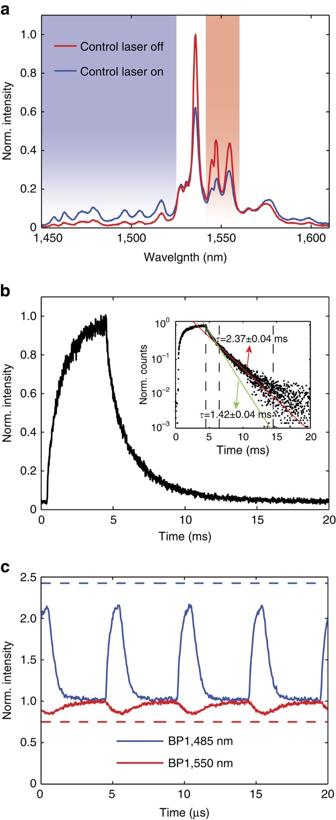Figure 4: Sub-lifetime modulation of Er3+light emission. (a) Experimental spectra for Er3+ions when VO2is in the insulating state (red) and in the metallic state (blue). (b) Decay trace of the time-resolved photoluminescence intensity from Er3+ions subjected to a pulsed 532 nm excitation. Inset shows lifetime fits, showing both fast (green) and slow (red) decay contributions with lifetimes ofand, respectively. (c) Time-resolved normalized photoluminescence of the Er3+ions in the multilayer structure when continuously pumped by a 532-nm laser while VO2is simultaneously switched by a pulsed 1,064 nm excitation at a 200 kHz repetition rate. Note the three orders of magnitude difference in the time-scale forcas compared withb. Blue and red solid lines represent two different spectral ranges of the bandpass (BP) filters (1,450–1,520 nm and 1,538–1,562 nm, respectively). The dashed lines show the theoretical maximum modulation calculated according to the spectra ina. Figure 4: Sub-lifetime modulation of Er 3+ light emission. ( a ) Experimental spectra for Er 3+ ions when VO 2 is in the insulating state (red) and in the metallic state (blue). ( b ) Decay trace of the time-resolved photoluminescence intensity from Er 3+ ions subjected to a pulsed 532 nm excitation. Inset shows lifetime fits, showing both fast (green) and slow (red) decay contributions with lifetimes of and , respectively. ( c ) Time-resolved normalized photoluminescence of the Er 3+ ions in the multilayer structure when continuously pumped by a 532-nm laser while VO 2 is simultaneously switched by a pulsed 1,064 nm excitation at a 200 kHz repetition rate. Note the three orders of magnitude difference in the time-scale for c as compared with b . Blue and red solid lines represent two different spectral ranges of the bandpass (BP) filters (1,450–1,520 nm and 1,538–1,562 nm, respectively). The dashed lines show the theoretical maximum modulation calculated according to the spectra in a . Full size image From the measured intrinsic rates ( Fig. 2c ) and the optical properties (that is, thickness and refractive index of individual layers), we can theoretically predict the normalized photoluminescence spectrum as a function of the VO 2 state (see Methods section and Supplementary Fig. 4 ). Using the measured refractive indices of VO 2 in the insulating state, as shown in Fig. 3c , the theoretical prediction (black line) matches well with the experimental spectrum without 1,064 nm laser illumination (shaded red area). For the insulating state, these calculations indicate that ∼ 70% of the total emission originates from MD transitions. Furthermore, as shown in Fig. 3d , when we use the measured refractive indices of VO 2 in the metallic state, we accurately predict the experimental spectrum obtained under 1,064 nm illumination. In the metallic state, the calculations suggest that MD transitions account for a much smaller percentage of emission ( ∼ 21%) and the vast majority of emission ( ∼ 79%) originates from ED transitions. Modulating spontaneous emission faster than lifetime limit We have therefore experimentally demonstrated that light emission from Er 3+ ions around 1.5 μm can be controllably switched from MD-dominant emission to ED-dominant emission. The result of this tuning is a significant modulation of the spectral shape, intensity and polarization of light emission. But the two most important implications of using a phase-change material to modulate light emission are the following: (i) The resulting modulation is broadband: in this experiment it covers the S-, C- and L-bands of conventional fibre-optic communication. Furthermore, given the ultra-broadband tuning of VO 2 refractive index ( Supplementary Fig. 5 ), the modulation range can easily be extended to shorter wavelengths (down to ∼ 500 nm). (ii) This all-optical switching exploits modifications to the LDOS rather than pumping on and off the electronic system governing light emission ( Supplementary Figs 6 and 7 ). There is a fundamental difference in the time-scales of these two processes. For example when Er 3+ ions are subjected to a pulsed excitation, the time-scale of the decay process is intrinsically limited by the long lifetime of the emitters. This is clearly evidenced in Fig. 4b , where full decay of photoluminescence from the 4 I 13/2 excited state requires almost 10 ms. On the other hand, if we use the 532 nm laser as a continuous excitation source and a pulsed 1,064 nm laser to dynamically switch the VO 2 phase, we can modulate the emission much faster than the decay time of Er 3+ . Figure 4c presents the normalized time-resolved photoluminescence in two wavelength ranges of interest: the S-band (1,450–1,520 nm; ED-dominant, blue line) and the C-band (1,540–1,560 nm; MD-dominant, red line) when the 1,064 nm control laser is chopped by an acousto-optic modulator (AOM) at a repetition rate of 200 kHz (see Fig. 2a for a schematic of the set-up and Methods for a detailed description of the measurements). We are able to clearly modulate light emission at time-scales more than three orders of magnitude faster than the lifetime of Er 3+ ions. (Note that without the VO 2 layer, no modulation is observed). In addition, we observe that when the S-band ED-emission (blue line) is enhanced, the C-band MD-emission (red line) is simultaneously suppressed: a clear indication that the modulated emission is consistent with the linked ED and MD LDOS changes. Note that the observed intensity modulation ratio of 2:1 results from our use of spectrally mixed ED and MD transitions. Even when switching from strongly MD emission (72% MD) to strongly ED emission (21% MD), the resulting intensity modulation will be lower than the average rate change (for example, 72%/21%), because ED and MD emission is mixed throughout the wavelength region of interest. One could achieve greater modulation depths by leveraging further differences beyond spectral intensity, such as the differing phase and polarization symmetries of ED and MD emission [22] . For example, the -phase shift between ED and MD transitions could be used for differential phase shift keying modulation [23] . We expect the fundamental limit on the speed of modulation to be significantly faster than this initial demonstration. In our experiment, the speed of switching is mainly limited by the AOM used to modulate the 1,064 nm control laser. In theory, dynamic modulation of emission through tuning the LDOS is only limited by retardation effects (that is, the time needed for light to propagate from the emitter to the reflecting layer and back). Therefore, the proposed device should allow modulation speeds approaching the time-scale of the IMT of VO 2 , which may be as fast as a few hundreds of femtoseconds [2] , [3] . The ultimate switching speed of our device could be tested in future studies by using an ultrafast laser (for example, Ti:Sapphire) to switch VO 2 (refs 2 , 4 ), while continuously pumping Er ions and monitoring their luminescence. Alternatively, one could electrically modulate the VO 2 layer to eliminate the need for ultrafast lasers and, in turn, investigate device performance in a more practical operating mode. Using phase-change media such as VO 2 to dynamically control spontaneous emission allows for complete device integration onto a single chip. Such a monolithic and heterogeneous integration is demonstrated here for the first time. Moreover, the use of phase-change materials dramatically increases the speed of LDOS modulation by orders of magnitude over initial mechanical approaches using piezoelectrically actuated mirrors [14] . Dynamic modulation of spontaneous emission in this monolithic nanoscale device could potentially reach ultrafast speeds, up to the phase transition kinetics of VO 2 . The presented device has a very simple geometry: it is composed of a stack of planar nanolayers. (See Supplementary Fig. 8 for demonstration of sub-lifetime modulation of Er 3+ emission using a different multilayer stack with a silicon spacer and gold mirror.) Although the respective thicknesses are crucial for engineering the modulation amplitude, there are no restrictions on the lateral dimensions. Indeed, in this experiment, both laser beams were confined to a diffraction-limited spot. Such a device could therefore easily be integrated on a variety of structures including cavities, waveguides and light-emitting devices. While this initial demonstration focused on all-optical modulation, switching of VO 2 could also be produced by electrically triggering the IMT [24] , [25] (see Supplementary Note 2 for discussion of switching energy). Combined with electroluminescent devices [26] , [27] , all-electrical direct modulation of emission could be obtained. The presented concept is not limited to Er 3+ ions and VO 2 . Indeed, the dynamic modulation of the LDOS could be extended to any phase-change material which experiences a large change in optical properties [1] , [5] , [7] , [28] and any emitters with spectrally close ED and MD transitions. Such emitters include both lanthanide [14] , [21] and transition-metal doped materials [29] , [30] that are widely used as phosphors in solid-state light sources. We therefore hope that the device and concept presented here will engage both academic and industrial researchers working on optoelectronics and nanophotonics. Device fabrication A 145-nm-thick Y 2 O 3 buffer-layer was deposited by e-beam evaporation followed by a 50-nm-thick Er 3+ :Y 2 O 3 thin-film emitter and covered by a ∼ 5-nm Y 2 O 3 layer. The sample was then annealed for 1 h at 900 °C under a flux of O 2 (0.5 lpm) to both activate the Er 3+ ions and crystallize the Y 2 O 3 . A TiO 2 spacer layer was subsequently deposited by reactively sputtering a pure titanium target under a controlled O 2 /Ar ratio (5%/95%). A low-temperature anneal (500 °C, 0.5 lpm O 2 ) was carried out to homogenize the TiO 2 layer. On top of this spacer layer, VO 2 was deposited by sputtering a V 2 O 5 target under a partial atmosphere of O 2 /Ar (0.08 sccm O 2 and 49.92 sccm Ar) while maintaining the substrate at 550 °C (ref. 24 ). Finally, a 200-nm silver layer was sputtered from a pure Ag target under an atmosphere of pure argon. All layer thicknesses, except the VO 2 layer, were monitored in situ using a quartz microbalance. All refractive indices and thicknesses were measured after deposition by ellipsometry. Experimental set-up The conventional photoluminescence spectrum of the sample was obtained using an inverted microscope in which an oil immersion ( × 100, 1.3 NA) objective was used for both excitation of the sample and collection of light emission. Er 3+ ions were pumped using a 532-nm frequency-doubled Nd:YVO 4 laser (Coherent Verdi). The laser line and emission from the sample were separated by a 665-nm dichroic mirror. The near-infrared emission was directed to an imaging spectrograph (IsoPlane SCT 320), subsequently dispersed (grating with 300 lines per mm blazed at 1.2 μm) and detected by a 2D InGaAs detector array (NIRvana, Princeton Instruments). Measured data have been corrected for the spectral and polarization dependence of the optical set-up using a calibrated quartz tungsten halogen lamp (Newport, Oriel 63355). For energy-momentum spectroscopy, a 100-mm Bertrand lens was used to image the back focal plane of the objective and thus project the radiation pattern of emission onto the entrance slit of the spectrograph. Using a rotatable polarizer, s - and p -polarized back focal plane spectra were then obtained by imaging the energy- and momentum-resolved photoluminescence on the 2D NIR camera. The all-optical modulation experiment was performed by focusing a 1,064-nm laser on the sample through the same × 100 objective. The laser line was filtered out by a 1,064-nm dichroic mirror and a 1,064-nm long pass filter. Precise coalignment of the 532 nm and the 1,064-nm lasers was enabled by using an eyepiece camera to monitor the position of their respective foci. Spectra of Er 3+ :Y 2 O 3 with VO 2 in the insulating and metallic states were obtained similarly to the photoluminescence set-up described above, by simply turning on and off the 1,064 nm laser. Time-resolved photoluminescence was acquired by a time-gated fiber-coupled InGaAs/InP single-photon avalanche photodiode, and a multichannel analyser (Stanford Research System 430) was used to build a histogram of photon arrival times. For conventional lifetime measurements of Er 3+ ions, the 532 nm laser was modulated by a mechanical chopper at a frequency of 38 Hz. Dynamic modulation of the LDOS through VO 2 switching was carried out by chopping the 1,064 nm laser with an AOM. Two long pass filters (1,350 nm and 1,450 nm) were cascaded (total OD 10) and systematically used to block the laser line at the entrance of the single-photon avalanche photodiode, and additional bandpass filters were used to measure specific wavelength ranges. Quantification of intrinsic emission rates To determine the intrinsic ED and MD emission rates, we measured the energy-momentum spectra of the Er 3+ :Y 2 O 3 emitter layer on quartz in a region without the TiO 2 /VO 2 /Ag overcoat layers ( Supplementary Fig. 1 ). With this technique, we measure the distribution of light emission from Er 3+ as a function of wavelength and in-plane momentum ( k || ). Using the procedure first described in Taminiau et al. [22] , experimental energy-momentum cross-sections in this three-layer system were fit to: where C is an overall scaling factor to account for experimental parameters that influence the number of measured counts but do not affect the radiation pattern. and are the normalized LDOS for a three-layer system calculated using equations in the Supplementary Information (S11–S14) of ref. 22 . (Note that the three-layer LDOS expressions may be readily derived from the five-layer system expressions provided in Supplementary Note 1 by setting n 0 = n 1 = n 2 =1). Using equation (1), we can fit the energy-momentum spectra to extract the spectrally resolved Einstein A coefficients ( A ED and A MD ). These coefficients, shown in Fig. 2c , represent the relative ED and MD intrinsic radiative rates at each wavelength, and are proportional to the intrinsic rates that one would expect in a homogeneous medium. Theoretical calculation of modified emission spectra To predict how the Er 3+ emission spectrum will be modified by the VO 2 phase-change, we use the measured intrinsic emission rates, and , inferred from the three-layer, emitter-on-substrate system together with the theoretically calculated LDOS for the five-layer device structure (described in Supplementary Note 1 ). The product of the intrinsic emission rate with the appropriate integrated LDOS yields the radiative decay rate for electric and magnetic transitions: where the LDOS is integrated in momentum over the range of values collected by the numerical aperture (NA) of our imaging system: and Note that in equations (4 and 5) we integrate over a line in momentum-space, which is consistent with the experimental set-up where the spectrum is collected after a Bertrand lens through a narrow slit spectrometer. The intensity of emitted light is proportional to the total emission rate, . Therefore, the theoretical normalized intensity can be calculated as follows: where I max and Γ max denote the maximum values of the light intensity and the total emission rate near 1.5 μm, respectively. Using equations (2, 3, 4, 5, 6), we can calculate the predicted emission spectrum of Er 3+ for both phases of VO 2 . As can be seen in Fig. 3c,d , there is an excellent agreement between the predicted and measured spectra. For reference, Supplementary Fig. 4 shows the calculated spectra (black line) decomposed into ED (shaded blue area) and MD (shaded red area) contributions. Simulation of branching ratios To quantify the fraction of light emission that originates from MD or ED transitions, we define branching ratios ( and ) as a function of the TiO 2 spacer layer thickness and VO 2 layer thickness : where is the phase-dependent refractive index of VO 2 . In our calculations, we use wavelength-dependent data for VO 2 at 25 and 95 °C measured by Jianing Sun of the J.A. Woollam Company to model the insulating and metallic phases, respectively ( Supplementary Fig. 5 ). For the complex refractive index of the silver layer, we use the Lorentz–Drude model in Rakić et al. [31] . How to cite this article: Cueff, S. et al. Dynamic control of light emission faster than the lifetime limit using VO 2 phase-change. Nat. Commun. 6:8636 doi: 10.1038/ncomms9636 (2015).